Isocitrate lyase mediates broad antibiotic tolerance inMycobacterium tuberculosis Mycobacterium tuberculosis (Mtb) is a persistent intracellular pathogen intrinsically tolerant to most antibiotics. However, the specific factors that mediate this tolerance remain incompletely defined. Here we apply metabolomic profiling to discover a common set of metabolic changes associated with the activities of three clinically used tuberculosis drugs, isoniazid, rifampicin and streptomycin. Despite targeting diverse cellular processes, all three drugs trigger activation of Mtb’s isocitrate lyases (ICLs), metabolic enzymes commonly assumed to be involved in replenishing of tricarboxylic acid (TCA) cycle intermediates. We further show that ICL-deficient Mtb strains are significantly more susceptible than wild-type Mtb to all three antibiotics, and that this susceptibility can be chemically rescued when Mtb is co-incubated with an antioxidant. These results identify a previously undescribed role for Mtb’s ICLs in antioxidant defense as a mechanism of antibiotic tolerance. Despite the advent of effective chemotherapy over 40 years ago, tuberculosis (TB) remains the leading bacterial cause of deaths due to a curable infection [1] . The causes of this shortfall are multifactorial. However, a key barrier to control of the TB pandemic is the limited number of chemotherapeutic agents effective against Mycobacterium tuberculosis (Mtb). Unlike most bacterial pathogens, Mtb exhibits an intrinsic resistance to most clinically approved antibiotics that has led to the need for months of multidrug therapy [2] . Mtb’s intrinsic resistance to most antibiotics has been traditionally ascribed to its unusually thick and hydrophobic envelope [3] , [4] . However, early studies by Nikaido and colleagues [5] , [6] established that although formidable, the limited permeability of the mycobacterial envelope was unlikely to fully explain this intrinsic resistance. Growing evidence has since identified a broader array of contributing factors that include the induction of antibiotic- and/or target-modifying enzymes and drug efflux pumps [3] . However, similar to most antibiotic mechanism-of-action studies, such studies have focused primarily around the primary drug–target interaction. Recent work has expanded the scope of physiologic factors associated with antibiotic resistance to include broader bacterial stress responses, such as the SOS DNA stress response, heat-shock response and oxidative stress response, as well as changes in metabolic state and activity [7] , [8] , [9] , [10] , [11] , [12] . These antibiotic-induced responses then contribute functionally to resistance. The specific mechanisms by which such factors mitigate against the consequences of primary antibiotic–target interactions remain incompletely defined. Here we sought to identify potential metabolic mediators of intrinsic resistance, or tolerance, to currently used TB drugs in replicating Mtb populations. Similar to other antibiotics, most TB drugs target a diverse array of cellular processes but share the common property of acting through biochemical targets. Metabolomics is the global study of metabolites in a biological system under a given set of conditions [13] . As metabolites are the biochemical currency of all biological processes, metabolomic approaches offer a direct and global biochemical window into the physiologic processes of a given cell, as well as the fates and actions of a given drug within the physiologic context of a viable cell [14] . We therefore applied a recently developed liquid chromatography–time of flight mass spectrometry platform to monitor antibiotic-induced changes in the pool size and turnover of Mtb’s endogenous metabolites associated with sublethal exposure to three clinically used TB drugs, isoniazid (INH), rifampicin (RIF) and streptomycin (STREP). All three drug treatments unexpectedly trigger a common pattern of metabolic alterations indicative of an activation of Mtb’s ICLs, enzymes commonly associated with assimilation of acetyl CoA and replenishment of tricarboxylic acid (TCA) cycle metabolites. Isogenic ICL-deficient Mtb strains exhibit a heightened sensitivity to all three antibiotics that can be rescued by co-incubation with either of the antioxidants thiourea or tempol. These findings thus reveal a previously undescribed function of Mtb’s ICLs in antibiotic tolerance that is mediated through a role in antioxidant defense rather than fatty acid metabolism. Distinct antibiotics elicit common metabolic responses Using a filter culture-based system and metabolomic profiling platform [14] , we first characterized the metabolomic response of Mtb to each of three mechanistically distinct TB drugs, RIF, STREP and INH ( Fig. 1 ). To do so, we exposed Mtb to bioequivalent doses of each drug (as determined by their minimum inhibitory concentrations (MICs) against Mtb grown atop agar-supported filters at larger inocula [15] suitable for metabolomic profiling ( Supplementary Fig. 1a ) and harvested samples during the pre-lethal phase of drug exposure. Although filter-based growth of Mtb precluded enumeration of colony-forming units (CFUs) as a measure of viability, pre-lethality was adduced by demonstrating the dose-dependent and kinetic reversibility of metabolic changes associated with drug treatment ( Figs 1 and 2 , and Supplementary Fig. 1b ) and withdrawal ( Fig. 3 and Supplementary Fig. 2 ), respectively, and observing no decrease in either total recoverable protein biomass or ATP levels ( Supplementary Fig. 3 ) on drug treatment. Drug-specific effects were then determined by comparing the relative abundances of 121 endogenous Mtb metabolites ( Fig. 1 and Supplementary Data 1 ). Although static measurements of metabolite pool sizes cannot strictly inform about flux through a given pathway, changes can be used to flag or screen for potential alterations in pathway activity. 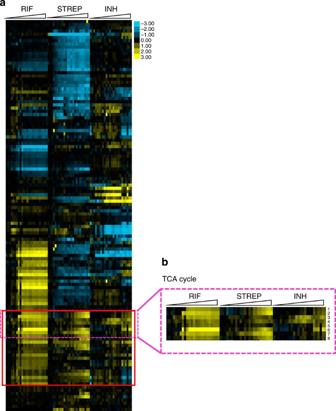Figure 1: Metabolic responses of Mtb strain H37Rv to antibiotic treatment. (a) Heat map profile depicting levels of 121 metabolites following drug treatments. Columns depict drug treatment as indicated, starting with untreated controls followed by antibiotic treatment with a dose range, increasing left to right, of 1 × to 64 × MIC. Rows indicate individual metabolites measured. Data were parsed using uncentred Pearson’s correlation with centroid linkage clustering and rendered using the image generation programme treeview (http://jtreeview.sourceforge.net/). Data are depicted on a log2scale relative to untreated control for each antibiotic. (b) Inset illustrating common TCA cycle metabolite responses to different antibiotics, and their associated pathways. Numbers on inset correspond to the following individual putative metabolites: 1. Succinate, 2. Fumarate, 3. Malate, 4. Pyruvate, 5. Hexose diphosphate, 6. Triose phosphate, 7. Deoxyribose phosphate, 8. Acetyllysine. RIF, rifampicin; STREP, streptomycin; INH, isoniazid. Figure 1: Metabolic responses of Mtb strain H37Rv to antibiotic treatment. ( a ) Heat map profile depicting levels of 121 metabolites following drug treatments. Columns depict drug treatment as indicated, starting with untreated controls followed by antibiotic treatment with a dose range, increasing left to right, of 1 × to 64 × MIC. Rows indicate individual metabolites measured. Data were parsed using uncentred Pearson’s correlation with centroid linkage clustering and rendered using the image generation programme treeview ( http://jtreeview.sourceforge.net/ ). Data are depicted on a log 2 scale relative to untreated control for each antibiotic. ( b ) Inset illustrating common TCA cycle metabolite responses to different antibiotics, and their associated pathways. Numbers on inset correspond to the following individual putative metabolites: 1. Succinate, 2. Fumarate, 3. Malate, 4. Pyruvate, 5. Hexose diphosphate, 6. Triose phosphate, 7. Deoxyribose phosphate, 8. Acetyllysine. RIF, rifampicin; STREP, streptomycin; INH, isoniazid. 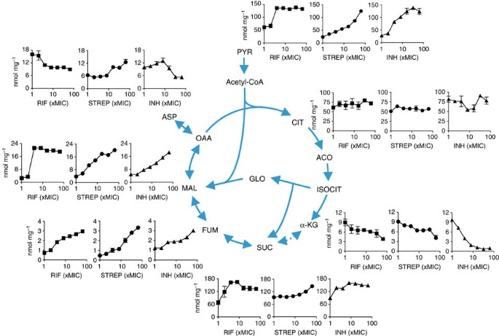Figure 2: Remodelling of Mtb TCA cycle with antibiotic treatment. Line graphs indicating levels of TCA cycle intermediates in H37Rv wild-type Mtb exposed to rifampicin (RIF), streptomycin (STREP) or isoniazid (INH). Pool sizes are expressed in nmol per mg protein (yaxis) over a bioequivalent range of antibiotic concentrations (xaxis) depicted as multiples of experimentally determined MIC values. All values are an average of three biological replicates±s.e. measured at 24 h (RIF and STREP) or 48 h (INH) post exposure. Results shown are the average of three biological replicates and are representative of a minimum of three independent experiments. αKG, α-ketoglutarate; ACO, aconitate; ASP, aspartate; CIT, citrate; FUM, fumarate; GLO, glyoxylate; ISOCIT, isocitrate; MAL, malate; OAA, oxaloacetate; PYR, pyruvate; SUC, succinate. Full size image Figure 2: Remodelling of Mtb TCA cycle with antibiotic treatment. Line graphs indicating levels of TCA cycle intermediates in H37Rv wild-type Mtb exposed to rifampicin (RIF), streptomycin (STREP) or isoniazid (INH). Pool sizes are expressed in nmol per mg protein ( y axis) over a bioequivalent range of antibiotic concentrations ( x axis) depicted as multiples of experimentally determined MIC values. All values are an average of three biological replicates±s.e. measured at 24 h (RIF and STREP) or 48 h (INH) post exposure. Results shown are the average of three biological replicates and are representative of a minimum of three independent experiments. αKG, α-ketoglutarate; ACO, aconitate; ASP, aspartate; CIT, citrate; FUM, fumarate; GLO, glyoxylate; ISOCIT, isocitrate; MAL, malate; OAA, oxaloacetate; PYR, pyruvate; SUC, succinate. 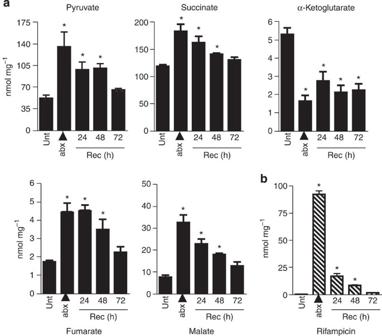Figure 3: Reversibility of antibiotic-induced changes in levels of TCA cycle intermediates. Abundance of TCA cycle intermediates (a) and antibiotic (b) in the wild-type Mtb strain H37Rv following removal from drug-containing plates. Bacteria were exposed to RIF for 24 h followed by transfer to drug-free plates. Recovery time points include 24, 48 and 72 h post transfer. Data are expressed as nmol mg−1normalized to protein content (yaxis);xaxis depicts conditions tested including untreated controls (unt), antibiotic exposure (abx) and time of recovery (24, 48 and 72 h). *Significant change (P<0.01) relative to untreated control by unpaired Student’st-test. Error bars represent s.e.m. of three biological replicates and all graphs are representative of a minimum of three independent experiments. Full size image Figure 3: Reversibility of antibiotic-induced changes in levels of TCA cycle intermediates. Abundance of TCA cycle intermediates ( a ) and antibiotic ( b ) in the wild-type Mtb strain H37Rv following removal from drug-containing plates. Bacteria were exposed to RIF for 24 h followed by transfer to drug-free plates. Recovery time points include 24, 48 and 72 h post transfer. Data are expressed as nmol mg −1 normalized to protein content ( y axis); x axis depicts conditions tested including untreated controls (unt), antibiotic exposure (abx) and time of recovery (24, 48 and 72 h). *Significant change ( P <0.01) relative to untreated control by unpaired Student’s t -test. Error bars represent s.e.m. of three biological replicates and all graphs are representative of a minimum of three independent experiments. Full size image Unsupervised hierarchical clustering analysis of drug-induced changes in metabolomes identified metabolite subsets common and unique to all three antibiotics. These subsets were then mapped to Mtb’s annotated metabolic network and analysed, using a hypergeometric distribution function, to identify statistically enriched or over-represented pathways. As shown in Table 1 , this analysis primarily identified pathways of central carbon metabolism, specifically the TCA cycle and glyoxylate metabolism, as well as the biosynthetic pathways for a number of amino acids. Given recent studies focused on the downstream consequence of the antibiotic–target interaction, we directed specific attention to effects on Mtb’s TCA cycle [16] . Table 1 Over-representation analysis of metabolic pathways altered with antibiotic treatment. * Full size table Antibiotics induce a specific remodelling of Mtb’s TCA cycle Irrespective of primary target or mode-of-action, all three antibiotics elicited similar accumulations of pyruvate, succinate, fumarate and malate, as well as decreases in α-ketoglutarate levels ( Fig. 2 ). As described above, these changes varied with the anti-mycobacterial dose, rather than potency, of antibiotics used. Levels of pyruvate, succinate and fumarate specifically increased two- to threefold, while levels of malate increased five- to sixfold and levels of citrate/isocitrate were unchanged. In addition, with the exception of α-ketoglutarate, all changes returned to near-baseline levels of untreated bacteria within the first 72 h (a maximum of three generation times under conditions of unrestricted logarithmic growth) after antibiotic withdrawal, although residual intrabacterial antibiotic levels were still present, supporting the pre-lethal nature of antibiotic exposure. ( Fig. 3a,b and Supplementary Fig. 2 ). The foregoing changes in the TCA cycle were indicative of an activation of Mtb’s isocitrate lyases (ICLs), which we investigated by quantitative reverse transcription PCR (qRT–PCR) analysis. Of the two annotated ICL genes in the H37Rv strain of Mtb , transcript levels of icl1 were increased 4- to 16-fold with antibiotic exposure, while levels of aceAa and aceAb (which encode the two segments of a second paralogous icl gene ( icl2 ) that has undergone a frameshift mutation in this strain) remained unchanged ( Fig. 4a ). Mtb’s ICLs serve dual roles in the glyoxylate shunt and methylcitrate cycles, pathways that play canonical roles in metabolism of even and odd chain fatty acids and/or branched chain ketoacids, respectively. Mtb’s ICLs have further been shown to be essential for both establishment and maintenance of infection in mice [17] , [18] , [19] . However, our studies, were conducted in the absence of a fatty acid carbon source, and thus suggested a non-canonical metabolic role for Mtb’s ICL in its response to antibiotic exposure. 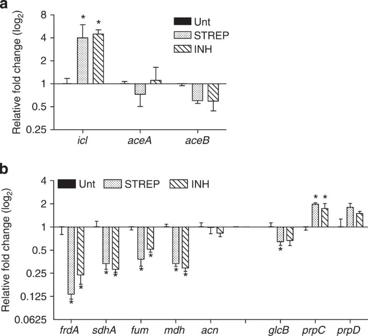Figure 4: Transcriptional response of Mtb metabolism to antibiotic exposure. (a) Expression of ICL genesicl1,aceAandaceBafter 24 h treatment with STREP or INH at 64 × MIC in wild-type Mtb strain H37Rv. Values are depicted relative to untreated controls (unt) on a log2scale. (b) qRT–PCR analysis of indicated TCA, glyoxylate and methylcitrate cycle genes after exposure to STREP or INH at 64 × MIC for 24 h in H37Rv Mtb. Values denote fold changes in mRNA levels relative to those of untreated controls (unt) and are depicted on a log2scale. For both figures, data are expressed as the average of three biological replicates±s.e. and are representative of a minimum of three independent experiments. *P<0.05 relative to respective untreated controls by unpaired Student’st-test. Figure 4: Transcriptional response of Mtb metabolism to antibiotic exposure. ( a ) Expression of ICL genes icl1 , aceA and aceB after 24 h treatment with STREP or INH at 64 × MIC in wild-type Mtb strain H37Rv. Values are depicted relative to untreated controls (unt) on a log 2 scale. ( b ) qRT–PCR analysis of indicated TCA, glyoxylate and methylcitrate cycle genes after exposure to STREP or INH at 64 × MIC for 24 h in H37Rv Mtb. Values denote fold changes in mRNA levels relative to those of untreated controls (unt) and are depicted on a log 2 scale. For both figures, data are expressed as the average of three biological replicates±s.e. and are representative of a minimum of three independent experiments. * P <0.05 relative to respective untreated controls by unpaired Student’s t -test. Full size image Broader qRT–PCR analysis of genes functioning in the interconnected network of TCA cycle, glyoxylate shunt, methylcitrate pathway and glycolysis/gluconeogenesis following treatment with INH or STREP revealed decreased transcript levels of frdA and sdhA , which encode enzymes catalysing the reversible conversion of succinate to fumarate. Levels of fum and mdh , which catalyse the interconversion of fumarate to malate and malate to oxaloacetate, respectively, were also decreased ( Fig. 4b ). These changes were matched by specific accumulations of succinate, fumarate and malate described above ( Fig. 2 ). Transcript levels for the methylcitrate cycle enzymes, prpC and prpD , in contrast, were increased ( Fig. 4b ), suggestive of a potential increase in flux not reported by a change in pool sizes of methylcitrate cycle intermediates, while transcript levels of acn , which encodes Mtb’s only annotated aconitase, and glcB , which encodes the terminal glyoxylate shunt enzyme, malate synthase, were largely unchanged ( Fig. 4b and Supplementary Fig. 4a ). These results thus revealed that antibiotics trigger a specific, but target—or mode-of-action—independent, metabolic response in Mtb that consists of a linked activation of its bifunctional isocitrate and methylisocitrate lyases, and net change in activity through the reductive arm of its TCA cycle. Treatment with RIF, an inhibitor of RNA polymerase and transcription initiation, resulted in widespread nonspecific decreases in transcript levels that precluded analogous analysis by qRT–PCR. ICLs mediate antibiotic induced remodeling of Mtb’s TCA cycle To evaluate the functional significance of the foregoing changes, we compared the metabolic response and survival of an ICL-deficient strain of Mtb to those of an isogenic wild-type counterpart and a genetically complemented strain following antibiotic challenge. Owing to the presence of a second paralogous ICL enzyme ( icl2 ) in the Erdman strain, which serves as the genetic background for the ICL-deficient strains used in this study, we first characterized the metabolomic responses of the wild-type Erdman strain to antibiotic treatment ( Supplementary Fig. 5 ), and confirmed the same alterations in TCA cycle intermediates observed in H37Rv strain ( Fig. 2 ). Of note, the genetically complemented strain used in these experiments (P icl1 ) expressed the icl1 gene under the control of a constitutive promoter at levels 64-fold higher than its wild-type counterpart and contained a STREP resistance cassette that also allowed this strain to serve as a drug-resistant control ( Supplementary Fig. 6a , blue bars). Metabolomic comparisons of wild-type, Δicl1/2 and the P icl1 complemented strains following treatment with bioequivalent doses of INH, STREP and RIF first confirmed that all strains accumulated antibiotics to similar levels, irrespective of ICL genotype ( Supplementary Fig. 1c,d ). These analyses next demonstrated that the previously described antibiotic-induced changes in TCA cycle-related metabolites, with the exception of α-ketoglutarate, were either attenuated or lacking in ICL-deficient Mtb ( Fig. 5a ), and restored for INH and RIF on genetic complementation with an extragenic wild-type allele of the icl1 gene ( Fig. 5a , blue bars). The persistently reduced levels of α-ketoglutarate in ICL-deficient Mtb on antibiotic treatment suggests the involvement of enzymes in addition to ICL. Consistent with its expression of a STREP resistance cassette, the genetically complemented Picl1 strain failed to exhibit these TCA cycle changes on treatment with STREP, but exhibited other metabolic responses to STREP, including an increase in fumarate, apparently independent of its antimycobacterial activity. Citrate/isocitrate levels, in contrast, increased on antibiotic treatment of ICL-deficient Mtb, likely to be reflecting its inability to redirect intermediates through the glyoxylate shunt ( Fig. 5a and Supplementary Fig. 4b ). 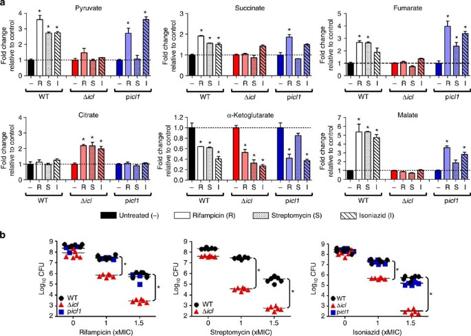Figure 5: Metabolic response and survival ofΔicl1/2-deficient Mtb mutant following antibiotic treatment. (a) Levels of TCA cycle intermediate in Erdman wild-type,Δicl1/2andpicl1-complemented strains exposed to antibiotic at 64 × MIC for 24 h (48 h for INH). Graphs depict fold changes in metabolite abundances relative to their respective untreated controls. Dashed lines indicate basal level of each intermediate for comparison. Data represent the average of three biological replicates±s.e. *P<0.05 relative to respective untreated control (−) by unpaired Student’st-test. (b) Survival of wild-type (black circles),Δicl1/2(red triangles) andpicl1-complemented (blue squares) strains exposed to antibiotic for 14 days. Viability was determined by measuring CFU ml−1counts, depicted on a log10scale (yaxis), for indicated antibiotic concentrations (xaxis). *P<0.05 in the comparison betweenΔicl1/2knockout and wild-type or complement by unpaired Student’st-test. Graph depicts variation between six biological replicates for each strain and is representative of three independent experiments. Figure 5: Metabolic response and survival of Δicl1/2- deficient Mtb mutant following antibiotic treatment. ( a ) Levels of TCA cycle intermediate in Erdman wild-type, Δicl1/2 and picl1- complemented strains exposed to antibiotic at 64 × MIC for 24 h (48 h for INH). Graphs depict fold changes in metabolite abundances relative to their respective untreated controls. Dashed lines indicate basal level of each intermediate for comparison. Data represent the average of three biological replicates±s.e. * P <0.05 relative to respective untreated control (−) by unpaired Student’s t -test. ( b ) Survival of wild-type (black circles), Δicl1/2 (red triangles) and picl1 -complemented (blue squares) strains exposed to antibiotic for 14 days. Viability was determined by measuring CFU ml −1 counts, depicted on a log 10 scale ( y axis), for indicated antibiotic concentrations ( x axis). * P <0.05 in the comparison between Δicl1/2 knockout and wild-type or complement by unpaired Student’s t -test. Graph depicts variation between six biological replicates for each strain and is representative of three independent experiments. Full size image qRT–PCR analysis revealed a similar pattern of ICL-dependent changes in TCA cycle gene expression following antibiotic treatment ( Supplementary Fig. 6b ). With the exception of frdA , the decreases in TCA cycle gene expression seen in antibiotic-treated wild-type Mtb were absent in the Δicl1/2 mutant. Consistent with its metabolic response, the STREP-resistant Picl1 strain showed minimal changes in gene expression on STREP exposure ( Supplementary Fig. 6b , blue bars). Phenotypic testing showed that ICL deficiency was accompanied by 100- to 1,000-fold increases in susceptibility to all three antibiotics over wild-type and ICL-deficient strains genetically complemented with a functional icl1 allele ( Fig. 5b ). These results thus establish that the previously described metabolic changes are triggered by the antimicrobial activities, rather than chemical properties, of the antibiotics tested, and are mediated by Mtb’s ICLs. Mtb’s ICLs mediate endogenous antibiotic tolerance In light of the apparent increase in glyoxylate shunt activity and decrease in activity through the reductive arm of the TCA cycle, we hypothesized that the foregoing changes might be indicative of an adaptive respiratory slowdown caused by an antibiotic-triggered increase in production of respiratory-derived reactive oxygen intermediates (ROIs). Using qRT–PCR, we monitored the expression of eight genes functionally characterized or annotated for their role in, or response to, oxidative and non-oxidative stresses in Mtb [20] , [21] . These included five genes specifically associated with protection against ROIs and reactive nitrogen intermediates (RNIs): furA , katG , trxB1 , ahpC and ahpD ; and three control genes associated with other stress responses including the dormancy transcriptional regulator dosR , as well as mbtB and hspX , which are induced in response to hypoxia, iron starvation and protein damage [22] , [23] , [24] . Treatment of wild-type Erdman Mtb with isoniazid or STREP resulted in induction of genes that can report exposure to ROI or RNI, including an eightfold increase in levels of furA , and three- to fourfold increases in levels of katG , trxB1 , ahpC and ahpD . Levels of dosR , mbtB and hspX , on the other hand, increased only slightly or were unchanged ( Fig. 6a ). 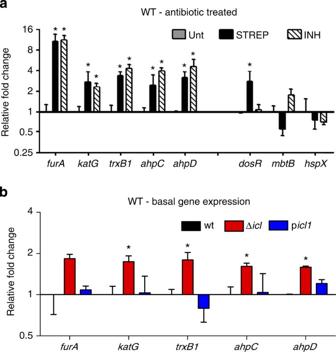Figure 6: Antibiotic-induced expression of stress response genes in Mtb. (a) qRT–PCR analysis of stress gene expression after exposure to 64 × MIC STREP or INH for 24 h in wild-type Mtb. (b) Basal expression of oxidative stress response genes in wild type,Δicl1/2andpicl1strains. Both graphs depict fold change in mRNA levels relative to untreated wild-type control (unt) and represent the average of three biological replicates±s.e. *P<0.05 in comparison with untreated wild-type control by Student’st-test. All data in this figure were generated in the Erdman Mtb strain background. Figure 6: Antibiotic-induced expression of stress response genes in Mtb. ( a ) qRT–PCR analysis of stress gene expression after exposure to 64 × MIC STREP or INH for 24 h in wild-type Mtb. ( b ) Basal expression of oxidative stress response genes in wild type, Δicl1/2 and picl1 strains. Both graphs depict fold change in mRNA levels relative to untreated wild-type control (unt) and represent the average of three biological replicates±s.e. * P <0.05 in comparison with untreated wild-type control by Student’s t -test. All data in this figure were generated in the Erdman Mtb strain background. Full size image We also found that basal expression levels all five ROI/RNI-responsive genes were 1.5- to 2-fold higher in ICL-deficient Mtb than in wild type, indicative of increased levels of endogenous oxidative/nitrosative stress in the absence of ICL ( Fig. 6b ). Complementation with the icl1 gene (p icl1 ) restored basal expression of these stress response genes back to wild-type levels with INH treatment ( Fig. 6b ). Treatment with antibiotics further increased the expression of these genes to levels higher than wild-type Mtb in the case of ahpC and ahpD ( Supplementary Fig. 7 ), while treatment of p icl1 complemented strains with STREP failed to elicit such changes. These data suggest that the foregoing antibiotic-induced metabolic changes are linked to an oxidative/nitrosative stress response in Mtb that is mitigated in part by activation of its ICLs. To elucidate the phenotypic significance of this response, we tested the effect of co-incubation with the thiol-based antioxidant thiourea [25] , on Mtb survival and gene expression following antibiotic treatment ( Fig. 7 and Supplementary Fig. 8a ). Thiourea did not exert a statistically significant effect on the survival of antibiotic-treated wild-type Erdman Mtb ( Fig. 7a ) but did, however, increase survival of STREP-treated, ICL-deficient Mtb by 10,000-fold, restoring survival to levels near that of STREP-treated wild-type cultures. As before, the Picl 1-complemented strain exhibited no changes in response to either STREP or thiourea, consistent with the presence of its plasmid-encoded STREP resistance cassette. Likewise, thiourea afforded 100- to 1,000-fold increases in CFU, approaching near-complete protection, in ICL-deficient Mtb treated with either RIF or INH ( Fig. 7a ). The radical scavenger Tempol (ref. 26 ) exerted similar, albeit weaker, effects in that it selectively improved survival of ICL-deficient, but not wild-type, Mtb following antibiotic treatment ( Supplementary Fig. 8a,c ). 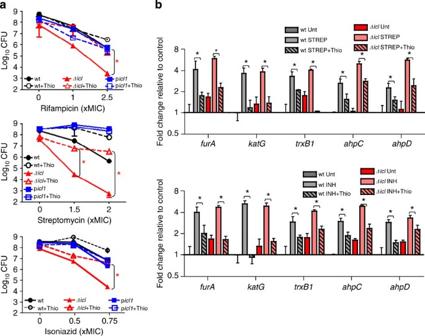Figure 7: Effect of thiourea on antibiotic tolerance and metabolism in Mtb. (a) Erdman wild-type (black),Δicl1/2(red) andpicl1-complemented (blue) strains were exposed to RIF, STREP or INH for 14 days in the presence (dashed lines) or absence (solid lines) of 10 mM thiourea. Survival was measured using colony-forming unit counts. Data depict the average of three biological replicates±s.e. on a log10scale, and are representative of a minimum of three independent experiments. *P<0.05 for the indicated comparisons by unpaired Student’st-test. (b) Relative mRNA levels of oxidative stress response genes in Erdman wild-type,Δicl1/2and picl1strains exposed to STREP or INH at 64 × MIC with (hatched bars) or without (solid bars) 100 mM thiourea for 24 h. mRNA levels are depicted relative to untreated wild-type control (unt) and represent the average of three biological replicates±s.e. Figure 7: Effect of thiourea on antibiotic tolerance and metabolism in Mtb. ( a ) Erdman wild-type (black), Δicl1/2 (red) and picl1- complemented (blue) strains were exposed to RIF, STREP or INH for 14 days in the presence (dashed lines) or absence (solid lines) of 10 mM thiourea. Survival was measured using colony-forming unit counts. Data depict the average of three biological replicates±s.e. on a log 10 scale, and are representative of a minimum of three independent experiments. * P <0.05 for the indicated comparisons by unpaired Student’s t -test. ( b ) Relative mRNA levels of oxidative stress response genes in Erdman wild-type, Δicl1/2 and p icl1 strains exposed to STREP or INH at 64 × MIC with (hatched bars) or without (solid bars) 100 mM thiourea for 24 h. mRNA levels are depicted relative to untreated wild-type control (unt) and represent the average of three biological replicates±s.e. Full size image Concurrent qRT–PCR-based profiling of the foregoing oxidative stress response genes confirmed that the phenotypically protective effects of both thiourea and Tempol were accompanied by matched decreases in transcript levels. For example, although addition of thiourea had no effect on the baseline expression of the stress response genes furA , katG , trxB1 , ahpC or ahpD in wild-type Erdman Mtb, treatment of ICL-deficient Mtb with thiourea reduced basal gene expression levels of these transcripts to wild-type levels in the absence of drug treatment ( Supplementary Fig. 8b ). Thiourea also caused a 50% decrease in the level of antibiotic-induced expression of ahpC , ahpD , trxB1 and furA , and near-complete suppression of katG induction in both wild-type and ICL-deficient Mtb ( Fig. 7b ). Neither thiourea nor tempol treatment had any effect on Mtb’s metabolic response to antibiotic treatment ( Supplementary Fig. 9 ). These data thus establish that Mtb’s ICLs mitigate against the bactericidal consequences of antibiotic-induced oxidative stress. Antibiotics are defined by their ability to suppress or kill bacteria. However, the factors that determine their activity remain poorly defined. Despite intensive focus on the primary drug–target interaction and its maladaptive consequences, knowledge of the endogenous mechanisms used by bacteria to resist antibiotic activity is incomplete and centred chiefly around mechanisms associated with the drug–target interaction, such as drug efflux pumps and antibiotic—and/or target—modifying enzymes [3] . However, growing evidence has implicated a broader range of physiologic factors [7] , [8] , [9] , [10] , [27] . Early studies on the mechanism of action of penicillin showed that non-growing bacteria were insensitive to the lytic effects of penicillin [28] . This insensitivity was found to be a property of many, if not all, antibiotic–bacteria pairs, termed tolerance, and was initially interpreted to reflect an apparent relationship between the rate of antibiotic-induced killing and rate of bacterial growth. More recent studies have begun to revise this view with the demonstration that even non-, or slowly, replicating bacteria could be rendered sensitive to antibiotics. Studies of Escherichia coli , Staphylococcus aureus and even Mtb have shown that the activity of many antibiotics: (i) is dependent on the activity of specific metabolic pathways, (ii) differs for replicating and non-replicating populations and (iii) can be dissociated from growth rate [7] , [12] , [27] . In Mtb , it was shown that adaptation to hypoxia was accompanied by a redirection of metabolic flux away from the TCA cycle and towards the generation of triglycerides, whose inhibition resensitized Mtb to antibiotics in absence of growth [7] . Such work has established antibiotic tolerance as an active cellular process rather than a passive consequence of slowed or arrested growth. Recent work has similarly revised the traditional view that antibiotics act exclusively through the inhibition of their primary targets, resulting in membrane damage, loss of cell wall integrity, or blockade of DNA replication or protein synthesis [16] . This view has been expanded to include the contribution of secondary effects such as the generation of ROI, although the origins and extent of their generation remain unresolved [25] , [29] , [30] . We found that sublethal exposures of Mtb to each of three different bactericidal TB drugs elicited a common and linked set of metabolic and, with the exception of RIF, transcriptional responses: activation of its ICLs and induction of oxidative stress response genes. Genetic deletion of its ICLs rendered Mtb >100-fold more sensitive to all three antibiotics in a manner that was accompanied by increases in both the basal and antibiotic-stimulated levels of expression of oxidative stress response genes. Moreover, both this heightened susceptibility and increased level of oxidative stress response gene expression could be restored to near-wild-type levels on co-incubation with either of two chemically unrelated antioxidants, thiourea (a redox-active thiol) or Tempol (a redox-shuttling nitroxide capable of catalytically detoxifying a wide range of ROI and RNI), at concentrations that did not affect growth [25] , [26] . Mtb’s ICLs thus participate in an endogenous metabolic defense against the bactericidal consequences of antibiotic-induced oxidative stress. The source(s) of putative antibiotic-triggered ROI and the mechanism(s) by which ICLs may defend against their bactericidal toxicity remain to be elucidated. ROI can arise as a byproduct of NADH-dependent electron flow through the metal, flavin and quinone co-factors of the respiratory chain, in particular complexes I and III [25] , [31] . Mutations that diminish fluxes through the TCA cycle have been reported to confer tolerance to bactericidal antibiotics [9] , [16] , [32] , suggesting a key role for respiration-derived ROI. In addition, a recent study reported that increased levels of a mitochondrial ICL-1 enzyme from Caenorhabtidis elegans resulted in decreased production of superoxide and increase in longevity, further supporting a key role for the glyoxylate shunt in regulating ROI production [33] . It will thus be of interest to determine the extent to which increased production of NADH, arising from inactivation of the glyoxylate shunt, may give rise to increased fluxes of ROI that might explain both the heightened susceptibility of ICL-deficient Mtb to the bactericidal antibiotics tested here and the palliative effects of thiourea and tempol. The foregoing studies identify a broad and metabolically encoded mechanism of in vitro antibiotic tolerance in Mtb mediated by its ICLs. ICL deficiency represents one of the most severely attenuating mutations of Mtb tested in a mouse model of TB [18] , [19] . Mtb’s ICLs catalyse only two known biochemical reactions, both of which use the same active site and play closely related roles in fatty acid metabolism [17] . Recent work reported the discovery of additional roles for ICL in adaptation to hypoxia and nutrient starvation that are unrelated to fatty acid metabolism but relevant to conditions thought to be encountered by Mtb in the host, while another study reported the discovery of a pathway closely interlinked with the glyoxylate shunt also involved in fatty acid metabolism termed the citramalate cycle [34] , [35] , [36] . Such evidence has thus begun to suggest that the profoundly attenuating effects of ICL deficiency in Mtb may reflect the loss of multiple physiologic functions, only some of which could be predicted by current genetic, bioinformatic and biochemical approaches. This current study now expands these to include an intrinsic mechanism of antibiotic tolerance in Mtb whose in vivo significance awaits future study. Mtb strains and culture Mtb strains were cultured in Middlebrook 7H9 broth media (Becton Dickinson, New Jersey) supplemented with 0.5 g l −1 Fraction V BSA, 0.05% Tyloxapol and 0.2% glucose as the primary carbon source. The wild-type Erdman strain was used as the control for all experiments using the Δicl1/2 and p icl1 strains, while the H37Rv strain was used as wild-type control for all other experiments [19] . For metabolomics experiments, Mtb was grown in liquid 7H9 to an optical density (OD 580 ) of 1 (5 × 10 8 cells per ml), 1 ml of culture then inoculated onto 0.22 μm nitrocellulose filters using vacuum filtration and placed on to 7H10 agar supplemented with 0.2% glucose. Mtb-inoculated filters were incubated at 37 °C for 5 days to generate sufficient biomass for subsequent metabolomic profiling. Filter-based assays for antibiotic and antioxidant treatments Bacteria grown on filters as described above were transferred to Middlebrook 7H10 plates (Becton Dickinson) containing control or antibiotics [14] , [37] . Antibiotic stocks were generated in dimethylsulphoxide or water and dissolved in 7H10 media to the appropriate concentrations. Antibiotic concentrations used were multiples of pre-determined MICs ( Supplementary Fig. 1a ) and included the following ranges: RIF: 0.1–6.4 μg ml −1 , STREP: 0.4–25.6 μg ml −1 , INH: 0.05–3.2 μg ml −1 . The antioxidants, thiourea (100 mM) and tempol (10 mM) dissolved in water, were added to 7H10 plates simultaneously with antibiotics as required. Concentrations of thiourea and tempol used were determined from survival assays for toxicity ( Supplementary Fig. 6a ). For recovery experiments, filters were first placed on antibiotic containing plates for 24 h, and then moved onto plates without antibiotic for the indicated time periods. Metabolite extraction Bacterial metabolism was quenched by immersing Mtb-laden filters into a solution of acetonitrile:methanol:water (40:40:20) precooled on dry-ice. Mtb removed from these filters in solution were mechanically lysed with 0.1 mm silica beads in a Precellys tissue homogenizer under continuous cooling at 2 °C. Samples were then clarified by centrifugation and the supernatant filtered through a 0.22-μm filter. Biomass of each sample was determined by measuring residual protein content using a colorimetric assay (Pierce BCA Protein Assay). Liquid chromatography–mass spectrometry Metabolites were separated using an Agilent 1200 LC system with a Cogent Diamond Hydride Type C column using a gradient of water and acetonitrile with 0.2% formic acid as previously described [14] . This system was coupled to an Agilent Accurate Mass 6220 TOF mass spectrometer and an isocratic pump was used for continuous infusion of a reference mass solution to allow mass axis calibration. Detected ions were classified as metabolites based on unique accurate mass–retention time identifiers for masses showing the expected distribution of accompanying isotopomers. Metabolites were identified using Agilent Quantitative Analysis software with a mass tolerance of <0.005 Da. Metabolite abundances were reported in relation to untreated vehicle control samples ( Supplementary Data 1 ) and, where indicated, quantified using a calibration curve generated from chemical standards spiked into control mycobacterial extracts to account for background lysate effects. Significantly altered metabolites (≥2-fold change in levels, P <0.05) were identified using Genespring Mass Profiler Professional software (Agilent Technologies) and pathway enrichment analysis was carried out using the online analytical tool Metaboanalyst ( www.metaboanalyst.ca ). With this approach, enriched pathways were identified using a hypergeometeric test based on a cumulative binomial distribution while also accounting for pathway interactions and interconnected nodes. Primary liquid chromatography–mass spectrometry data ( Supplementary Data 1 ) are deposited in the Dryad Digital Repository ( http://dx.doi.org/10.5061/dryad.kd8cj ). MIC and CFU assays Experimental MICs were determined using 24-well plates. Wells were filled with 7H10 media containing a range of drug concentrations. Ten microlitres of Mtb at an OD 580 of 1 (5 × 10 8 cells per ml) was added to each well and plates were incubated at 37 °C for 3 weeks. The minimal antibiotic concentration that completely suppressed bacterial growth was determined to be the experimental MIC. CFU growth assays were conducted in 96-well plates. Bacteria were diluted to an OD 580 0.1 (5 × 10 7 cells per ml) in 7H9 in each well. Antibiotics and other supplements were added at indicated concentrations and incubated for 2 weeks. Bacterial cultures were then serially diluted and plated on 7H9 agar plates, incubated for 3 weeks at 37 °C and colonies counted by hand. RNA extraction and qRT–PCR analysis Mtb was grown on filters and exposed to antibiotic treatments as described above. Bacteria were scraped off filters into TRIZOL solution and mechanically lysed with 0.1 mm silica beads in a Precellys tissue homogenizer. Lysates were clarified by centrifugation and TRIZOL supernatant removed and used for RNA extraction. RNA was isolated using a Qiagen RNA extraction kit. RNA concentrations were determined using a Nanodrop. qRT–PCR reactions were conducted using a SYBR-Green one-step kit (BioRad) and analysed using a Roche Lightcycler 480 II instrument. C T values were internally normalized to sigA transcript levels and depicted as log 2 values relative to untreated controls. Primer sequences are included in Supplementary Data 2 . Accession codes: Primary LC–MS data are deposited in the Dryad Digital Repository under doi:10.5061/dryad.kd8cj ( http://dx.doi.org/10.5061/dryad.kd8cj ). How to cite this article: Nandakumar, M. et al. Isocitrate lyase mediates broad antibiotic tolerance in Mycobacterium tuberculosis . Nat. Commun. 5:4306 doi: 10.1038/ncomms5306 (2014).